A pistil-expressed pectin methylesterase confers cross-incompatibility between strains ofZea mays A central problem in speciation is the origin and mechanisms of reproductive barriers that block gene flow between sympatric populations. Wind-pollinated plant species that flower in synchrony with one another rely on post-pollination interactions to maintain reproductive isolation. In some locations in Mexico, sympatric populations of domesticated maize and annual teosinte grow in intimate associate and flower synchronously, but rarely produce hybrids. This trait is typically conferred by a single haplotype, Teosinte crossing barrier1-s . Here, we show that the Teosinte crossing barrier1-s haplotype contains a pistil-expressed, potential speciation gene, encoding a pectin methylesterase homolog. The modification of the pollen tube cell wall by the pistil, then, is likely a key mechanism for pollen rejection in Zea and may represent a general mechanism for reproductive isolation in grasses. Reproductive isolation is essential for the origin of new species [1] . Wind-pollinated plant species, like those of the grass family, rely on post-pollination barriers to prevent hybrid production, including both pollen–pistil interactions that prevent fertilization and post-fertilization hybrid abortion or sterility [2] , [3] , [4] . Maize ( Zea mays ssp. mays ) was domesticated from annual teosinte ( Z. mays ssp. parviglumis ) in the Balsas River valley of Mexico about 9000 years ago [5] . Despite this recent divergence and the full compatibility of some maize and teosinte populations, other sympatric populations of annual teosinte grow together and flower synchronously with domesticated maize, but rarely produce hybrids [6] , [7] . The Teosinte crossing barrier1-s ( Tcb1-s ) haplotype, originally identified from strains of Z. mays ssp. mexicana teosinte, confers this cross-incompatibility trait to these plants. In Z. mays , haplotypes at three loci, Tcb1-s , Gametophyte factor1-s ( Ga1-s ) and Gametophyte factor2-s ( Ga2-s ) confer unilateral cross-incompatibility against varieties carrying the tcb1 (or ga1 or ga2 , respectively) haplotype. While Ga1-s and Ga2-s are widespread in domesticated maize, Tcb1-s is almost exclusively found in wild teosinte populations, with the exception of one ancient Maiz Dulce sweet corn variety from Mexico [8] . Tcb1-s was first described in teosinte subspecies mexicana Collection 48703 from central and southern Mexico [6] , [7] , [9] . Other collections of teosinte of both mexicana and parviglumis subspecies from the central Mexican plateau also carry Tcb1-s [10] . Since Tcb1-s is unilateral it can be crossed into maize and functions as it does in teosinte to reject standard maize pollen [7] . Tcb1-s females block fertilization by maize ( tcb1 type) pollen by restricting pollen tube growth in the pistil (silk) [4] . This function makes Tcb1 a candidate speciation gene contributing to isolation of diverging maize and teosinte populations, as wild teosinte populations respond to the pressure of cultivated, closely related varieties of domesticated maize [10] . In the reciprocal cross, teosinte pollen is able to fertilize maize, although at a slight disadvantage when in competition with maize pollen [7] . The Tcb1-s locus contains male ( Tcb1-male ) and female ( Tcb1-female ) genes, which are tightly linked but separable by recombination [4] . 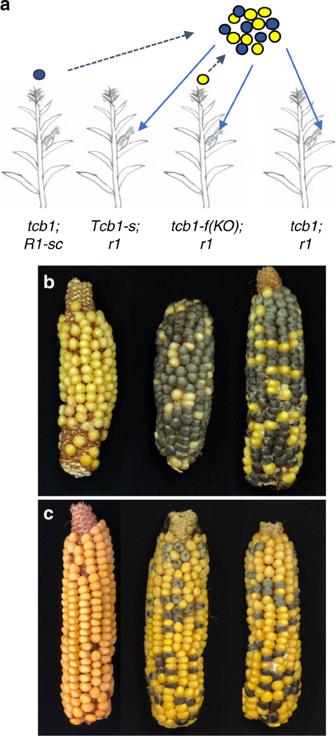Fig. 1 Mixed pollination test of theTcb1-fmutants.aScheme of the experiment: Two pollen donor lines and three pollen receiver lines were used. Pollen from atcb1; R1-self colormaize line (purple circles), produces purple kernels, while pollen from test plants (yellow circles) produces white or yellow kernels. Pollen from the two donors was mixed and put on three receiving ears: (1)Tcb1-sears to verify theTcb1-malefunction from theKOline; (2)tcb1-f(KO)ears to test the presence/absence of the female barrier in the knockout mutant individuals; and (3) a maize (tcb1; r1) neutral ear to identify the ratio of viable pollen grains from the two donors in the mixture.bEars from the three pollen recipients for thetcb1-f(KO1)) test.cEars from the three pollen recipients for thetcb1-f(KO2)test. In both tests, pollen from theKOplants successfully fertilized theTcb1-sear (left ear inbandc), while the ears fromKOplants showed no barrier totcb1maize pollen with a similar frequency of purple kernels on mutant ears and the neutral test ears (middle and right ears inbandc) Thus, there are four functional haplotypes at this locus (Supplementary Table 1 for gene content and origin): Tcb1-s has both functional male and female genes, Tcb1-m has only the functional male gene [4] , [10] , Tcb1-f has only the functional female gene, and the tcb1 haplotype found in almost all maize lines has neither of the two functional genes. In teosinte, Tcb1-f activity in the silks prevents fertilization by maize ( tcb1 ) pollen, while Tcb1-m activity in pollen enables fertilization of Tcb1-f or Tcb1-s females [4] . There are two alternative explanations of rejection of tcb1 pollen: (1) tcb1 pollen expresses an allele of Tcb1-m that is recognized by the Tcb1-female gene leading to directed inhibition of tcb1 but not the unrecognized Tcb1-m pollen; or (2) Tcb1-m confers a function to pollen not present in tcb1 allowing it to overcome the barrier set up indiscriminately in Tcb1-f pistils. This second case is preferred since pollen heterozygous for Tcb1- s and tcb1 haplotypes (using a trisomic line carrying a duplication of the short arm of Chromosome 4) fertilizes Tcb1-s females, indicating that the Tcb1-female : Tcb1-male match overcomes the Tcb1-female : tcb1-male mismatch (the situation is similar for the Ga1 and Ga2 systems) [11] , [12] . This study demonstrates that the Tcb1-female gene encodes a pistil-expressed pectin methylesterase38 (PME38) homolog. The identity of this gene suggests a mechanism for reproductive isolation in diverging plant populations of maize and some teosintes, in which the pollen tube cell wall is modified by the female thus preventing continued pollen tube growth and delivery of the sperm cells. Agriculturally, this work may facilitate reproductive isolation of specialty crops, and enrichment of crop plant germplasm by overcoming barriers to crossing with wild relatives [13] . Fine mapping analysis and mutant screen of Tcb1-s To clone the Tcb1 genes, fine mapping of Tcb1-s::Col48703 haplotype was performed based on a tcb1 backcross population of ~15,000 chromosomes. Using the maize B73 genome as a reference [14] , the Tcb1 locus was delimited to a region spanning 480 kb on the short arm of Chromosome 4. Within this region, there are 10 annotated genes. 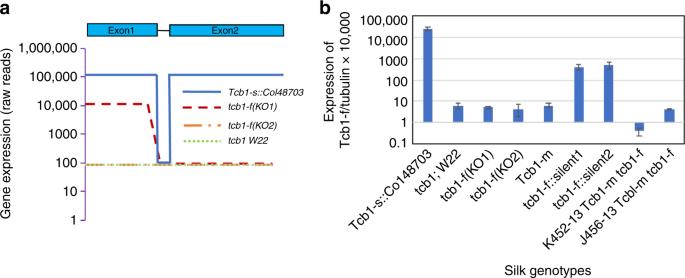Fig. 2 Gene expression profiling identifies aPME38as aTcb1-fcandidate gene. RNA samples collected from silks of different genotypes was analyzed by RNA-Seq and RT-PCR.aTcb1-f/PME38gene structure is shown above the graph (solid line indicates single intron), and RNA-Seq read depth is shown for theTcb1-f/PME38gene.bTcb1-f/PME38gene expression, compared totubulinlevels as a control, as measured by qRT-PCR inTcb1-s and loss-of-functionTcb1-slines:Tcb1-s, full strengthTcb1-sbarrier line;tcb1-f(KO1)andtcb1-f(KO2), two loss-of-function alleles from aMutatortransposon mutagenesis;Tcb1-m, a spontaneousTcb1-maleonly line;tcb1-f::silent lineage1andtcb1-f::silent lineage2; andK452-13andJ456-13, twoTcb1-maleonly lines that lostTcb1-fby recombination. Error bars equal the standard error of the mean. Source data for RT-PCR are provided as a Source Data file. RNA-seq reads provided in NCBI BioProject PRJNA528983 However, all of these were ruled out as candidates for Tcb1 functions because they either had identical sequence with identical expression levels between tcb1 and Tcb1-s haplotypes or no expression in the silk or pollen in Tcb1-s or tcb1 (mapping markers included in Supplementary Table 2 ). The Tcb1 genes, therefore, are likely absent from the maize genome. This is not surprising considering the widespread structural variations in genomes between maize lines and between teosinte populations [15] . Using gene content information from B73, clones were isolated and sequenced from a Bacteria Artificial Chromosome (BAC) library of the Tcb1-s::Col48703 haplotype to identify gene models present in the Tcb1-s haplotype that are absent in maize reference genomes. These BACs were assembled into three contigs with two gaps in the Tcb1-s region. Four new gene models from this assembly could be eliminated as candidates based on lack of expression or identical sequence coupled with identical expression to unlinked maize genes. However, the data did provide more mapping markers for delineating the Tcb1-f and Tcb1-m gene regions. To identify Tcb1-f knockout mutants, maize lines homozygous for the Tcb1-s::Col48703 haplotype and carrying active Mutator transposons were crossed to maize inbred A195 su1 . The progeny are expected to be heterozygous for Tcb1-s with su1 ~6 cM away and in repulsion [7] . Due to the rejection of the tcb1 pollen (which is predominantly su1 ), about 3% of the kernels in every ear with functional Tcb1-f were expected to be su1 homozygotes in this open-pollinated population, while any ears without a crossing barrier that fail to exclude tcb1 pollen were predicted to segregate su1 at 25%. Out of a population of ~6000 individuals, two exceptional ears were found. One ear segregated for 25.6% sugary. This allele is termed tcb1-f(KO1) . The second isolate contained a sector of about 45 kernels within which the segregation was one-fourth sugary despite sugary segregating at ~3% over the rest of the ear. This allele is termed tcb1-f(KO2) and was recovered from the loss-of-function sector. Mixed pollination tests with the progeny of both individuals show that the loss of function is heritable, and both variants fertilized a Tcb1-s/tcb1 strain normally, indicating the retention of the male function of Tcb1-s ( Tcb1-f mutated, but Tcb1-m intact) (Fig. 1 ). In the case of tcb1-f(KO2) , progeny of seeds within the loss-of-function side of the ear inherited the knock-out, while those on the other side of the ear inherited fully functional Tcb1-s . Fig. 1 Mixed pollination test of the Tcb1-f mutants. a Scheme of the experiment: Two pollen donor lines and three pollen receiver lines were used. Pollen from a tcb1; R1-self color maize line (purple circles), produces purple kernels, while pollen from test plants (yellow circles) produces white or yellow kernels. Pollen from the two donors was mixed and put on three receiving ears: (1) Tcb1-s ears to verify the Tcb1-male function from the KO line; (2) tcb1-f(KO) ears to test the presence/absence of the female barrier in the knockout mutant individuals; and (3) a maize ( tcb1; r1 ) neutral ear to identify the ratio of viable pollen grains from the two donors in the mixture. b Ears from the three pollen recipients for the tcb1-f(KO1) ) test. c Ears from the three pollen recipients for the tcb1-f(KO2) test. In both tests, pollen from the KO plants successfully fertilized the Tcb1-s ear (left ear in b and c ), while the ears from KO plants showed no barrier to tcb1 maize pollen with a similar frequency of purple kernels on mutant ears and the neutral test ears (middle and right ears in b and c ) Full size image Tcb1-female encodes a PME38 homolog RNA from silks of four genotypes were subjected to short read RNA-seq: the two knockout mutants, a standard maize inbred line W22 (genotype tcb1 ), and a functional Tcb1-s line (a W22 subline to which the Tcb1-s::Col48703 haplotype had been introduced by backcrossing). Transcript models were assembled de novo from the RNA-seq reads, and expression levels of genes were compared between lines. One gene, encoding a maize PME38 homolog, was identified as a candidate for the Tcb1-f gene. This gene is highly expressed in Tcb1-s silks (with a peak read depth of ~100,000) compared to the standard maize tcb1 W22 silks, tcb1-f(KO2) silks (maximum read depths of ~100) and tcb1-f(KO1) silks (maximum read depth of ~10,000 for the 5′ end and ~100 for the 3′ end of the transcript model) (Fig. 2a ). qRT-PCR confirmed this expression difference (Fig. 2b ). A BAC clone from the Tcb1-s library carrying this PME38 homolog was identified by PCR. By comparing mRNA and BAC sequences, a 99-base pair intron was identified in Tcb1-f (Supplementary Fig. 1 ). Comparison of this gene to maize sequences (maizegdb.org and NCBI) by BLAST demonstrated that it is not present in the maize B73 reference genome, which is consistent with the mapping data. Its closest homologs are pseudogenes located at the ga1 locus in both B73 and W22 and a silk-expressed (putative Ga1-f ) gene in Ga1-s maize [16] . It is likely that the small number of reads from tcb1 RNA-Seq that map to the gene are a consequence of miss-assignment of reads from the poorly expressed pseudogenes. Fig. 2 Gene expression profiling identifies a PME38 as a Tcb1-f candidate gene. RNA samples collected from silks of different genotypes was analyzed by RNA-Seq and RT-PCR. a Tcb1-f/PME38 gene structure is shown above the graph (solid line indicates single intron), and RNA-Seq read depth is shown for the Tcb1-f/PME38 gene. b Tcb1-f/PME38 gene expression, compared to tubulin levels as a control, as measured by qRT-PCR in Tcb1- s and loss-of-function Tcb1-s lines: Tcb1-s , full strength Tcb1-s barrier line; tcb1-f(KO1) and tcb1-f(KO2) , two loss-of-function alleles from a Mutator transposon mutagenesis; Tcb1-m , a spontaneous Tcb1-male only line; tcb1-f::silent lineage1 and tcb1-f::silent lineage2 ; and K452-13 and J456-13 , two Tcb1-male only lines that lost Tcb1-f by recombination. Error bars equal the standard error of the mean. Source data for RT-PCR are provided as a Source Data file. RNA-seq reads provided in NCBI BioProject PRJNA528983 Full size image In addition to the two knockout mutants above, several other lines derived from Tcb1-s::Col48703 have lost female barrier function. One was recovered during early backcrossing of the Tcb1-s::Col48703 haplotype into maize [6] . Mixed pollination confirmed this is a Tcb1 - male only plant (Supplementary Fig. 2 ). Additionally, two independent Tcb1-s lines were isolated in which the barrier gradually lost strength over 10 generations of backcrossing to maize [4] , and are named as tcb1-f::silent lineage1 ( tcb1-f::sl1 ) and tcb1-f::silent lineage2 ( tcb1-f::sl2 ), based on the progressive manner of the barrier loss. This PME38 has much lower expression in these three lines than Tcb1-s::Col48703 (Fig. 2b ). Expression of the PME38 was also tested on two Tcb1-m lines from the mapping population, which lost the Tcb1-female gene by recombination. Again, the PME38 expression was much lower than in Tcb1-s lines (Fig. 2b ). A PCR-based derived Cleaved Amplified Polymorphic Sequence (dCAPS) marker was designed for the PME38 gene (Supplementary Fig. 3 ). This marker was tested on the 15 closest recombinants from the mapping population of ~15,000 individuals (including four recombinants between the Tcb1-f and Tcb1-m genes) [4] . Of the 15 plants, 6 carried Tcb1-f and blocked maize pollen, and 9 lacked the barrier. Results showed that all the six recombinants that carry the barrier had the PME38 gene, while in all nine recombinants that are receptive to maize pollen, this PME38 was absent, demonstrating tight linkage between the PME38 and Tcb1-f barrier function. RNA-seq data suggest that the mutation in the PME38 lies in the first exon in tcb1-f(KO1) (Fig. 2a ). Quite differently, in tcb1-f(KO2) mutant silk RNA-seq reads had the same low level of expression as tcb1 silks along the whole PME38 transcript, and the whole coding of PME38 can be PCR-amplified from tcb1-f(KO2) genomic DNA but not tcb1-f(KO1) (Supplementary Fig. 4 ). Whole genome resequencing of both mutants identified a Hopscotch retrotransposon insertion in the first exon in tcb1-f(KO1) , a mutation unrelated to Mutator transposons, but deletions and non- Mutator insertions occur in these lines [17] . This insertion is close to the site where the PME38 expression drops sharply. PCR spanning both ends of the insertion confirmed the insertion event and the border sequences (Supplementary Fig. 5 ). In contrast, in tcb1-f(KO2) , the PME38 gene was fully assembled, consistent with the PCR data. The tcb1-f(KO2) allele then could either be mutated in a regulatory region, potentially hundred kilobases away from the coding region, or could be an epi-allele. Similarly, no mutations were found in the coding region in the Tcb1-m line or the tcb1-f::sl1 or tcb1-f::sl2 lines described above. Reversion of silenced tcb1-f loss-of-funtion lines Since several of the loss-of-function lines did not carry mutations in the PME38 coding region, tests were performed to determine if they might be epi-alleles and so could revert back to full-strength Tcb1-s . The tcb1-f(KO2) , tcb1-f::sl1 , and tcb1-f::sl2 lines were tested for reversion to Tcb1-s in double mutants with the mediator of paramutation1 ( mop1 ) mutation. MOP1 encodes a RNA-dependent RNA polymerase and is a key component of RNA-directed DNA methylation [18] . mop1 mutations reactivate silenced genes and affect broad developmental programs [19] . Re-activation of the Tcb1-f function was rare. In only ~14–22% of the mop1 females tested, did the loss-of-function plants show some recovery of Tcb1-f function. Pollen competition experiments were performed for full strength, wild-type Tcb1-s females, tcb1 females, and the tcb1-f loss of function lines without sequence changes ( tcb1-f(KO2) , tcb1-f::sl1 , tcb1-f::sl2 , and a few Tcb1-m ) (Fig. 3 and Source Data file). All of the Tcb1-s ears tested showed strong preference for Tcb1-s pollen (0–7% kernels from tcb1 pollen regardless of the ratio of the two pollen types in the mix as indicated by the neutral ear) with the kernel ratio on the test ear and control ear being different from each other at p < 0.0001 (two-tailed Fisher exact test) (Fig. 3b ). Of the 36 mop1; tcb1-f loss of function females tested only one ( tcb1-f::sl1 ; mop1 ) had as strong of a pollen preference as full strength Tcb1-s females, but five had a difference between the test and control ears at p < 0.0001 and an additional three females could be included if the stringency was relaxed to p < 0.01 (two-tailed Fisher exact test) (Fig. 3b ). These partial revertants included plants of lines tcb1-f(KO2) , tcb1-f::sl1 , and tcb1-f::sl2 . Of the 12 loss of function plants tested that were heterozygous wild-type for mop1 , none of the plants passed the more stringent p < 0.0001 threshold and one passed the less stringent p < 0.01 threshold (two-tailed Fisher exact test). Additionally, none of the 13 comparisons between two tcb1 ears had significant differences between the two ears. Fig. 3 Reversion of tcb1-f loss-of-function. a Revertant ear (marked by asterisk in b and c ) pollinated by a mix of tcb1; R1-sc and Tcb1-m ; r1 pollen showing higher frequency of yellow kernels on the test ear than the tcb1 control ear. b Results of mixed pollination tests on four genotypes: tcb1 , Tcb1-s , tcb1-f ( loss-of-function(lof)) alleles, and tcb1-f(lof) mop1 double mutants. The percentage of kernels from tcb1 pollen on the test ear are plotted on the x -axis and the percentage of kernels from tcb1 pollen on the control tcb1 ear on the y -axis. Equal percentages in the two ears indicates no barrier (line with slope = 1). Red circles indicate ears with significantly fewer tcb1 kernels in the test ear vs. the control ear at p < 0.0001 and blue circles at 0.0001 < p < 0.01 (two-tailed Fisher exact test). The loss-of-function line is indicated for each revertant. c Tcb1-f/PME38 gene expression level and barrier strength. Barrier strength is expressed as the ratio of kernels from Tcb1-s vs. tcb1 pollen on the test ear vs. the control tcb1 ear (columns), with a fraction of 1.0 indicating no barrier and significantly higher values a functional barrier. Tcb1-f/PME38 RNA levels are expressed as relative to the tubulin control gene (orange line). Error bars in c equal the standard error of the mean. Individual pedigree numbers are given for loss-of-function plants tested for reversion in a and c . Source data for panels b and c is provided in a Source Data file Full size image A subset of homozygous mop1 tcb1-f::sl2 plants were tested at random for PME38 expression in silks prior to pollination. Among the seven tested plants, one plant, yx57-13, showed increased expression, about 400-fold higher expression compared to that of the standard W22 maize and eight times higher than tcb1-f::sl2 plants (Fig. 3c ). This plant was the only one of the seven tested for expression that recovered the ability to reject tcb1 pollen, although not as efficiently as full strength Tcb1-s plants, which have still higher expression of the PME38 gene. This indicates a correlation between PME38 expression level and the female barrier strength with the expression level in tcb1-f::sl1 and tcb1-f::sl2 being below the expression threshold for producing a detectable barrier. This correlation and the Hopscotch insertion in tcb1-f(KO1) supports this PME38 as the Tcb1-f gene. In addition to the Tcb1-s::Col48703 strain descried above, three other teosinte-derived Tcb1-s lines, two from ssp. mexicana and one ssp. parviglumis [10] , were tested for Tcb1-f/PME38 expression in silk tissue. In all three lines, Tcb1-f/PME38 expression levels are extremely high and comparable to that of the original central plateau TIC haplotype Tcb1-s::Col48703 (Fig. 4 ). Interestingly, even though none of the modern north American maize lines tested to date carry the Tcb1-s haplotype, Tcb1- s was identified in lines descended from an ancient Maiz Dulce variety, Jalisco78 that grows at intermediate altitudes in southwestern Mexico, during a survey for cross-incompatibility factors [8] . This is a specialty line that may have undergone selection for cross-incompatibility factors similarly to Ga1-s in maize popcorn lines but in this case to maintain a sweet corn trait. Whether this Maiz Dulce line acquired Tcb1-s from nearby teosinte populations during its origin is unknown, but maize lines from this region have been shown to have substantial introgression from ssp. mexicana teosintes [20] . Fig. 4 Mean expression of Tcb1-f/PME38 in lines with different Tcb1-s haplotypes. W22 is a standard maize tcb1 line, Tcb1-s::Col48703 , Tcb1-s::Col109-4a , and Tcb1-s::Col207-5d are three independent collections of Zea mays ssp. mexicana tesointe lines; Tcb1-s::Col104-4a , a Zea mays ssp. parviglumis line; and DGF1222-2 derived from Maiz Dulce, an ancient Mexican maize sweet corn variety [8] . Error bars equal the standard error of the mean. Source data for RT-PCR are provided as a Source Data file Full size image Diversity and relationship of Tcb1-f to other PME genes Predicted Tcb1-f/PME38 coding sequences are identical in all five Tcb1-s lines: three mexicana accessions, one parviglumis accession, and the Maiz Dulce line. One single nucleotide polymorphism (SNP) in the intron separates these lines into two groups: one group including the parviglumis line (Col104-4a) and one mexicana line (Col109-4a), and the other group including two mexicana lines (Col48703 and Col207-5d) and the Maiz Dulce line (Supplementary Fig. 6 ). The most similar gene to Tcb1-f/PME38 is a candidate PME gene for Ga1-female function. This gene, termed ZmPME3 , was found to be expressed in the silks of Ga1-s , but not in ga1 silks, and maps to the Ga1 locus [16] . Alignment of the ZmPME3 and Tcb1-f/PME38 show that the two PMEs differ in eight amino acids (Supplementary Fig. 7 ). The number of polymorphisms (15 of 1296 nucleotides) between Tcb1-f/PME38 and ZmPME3 suggests that these two genes diverged ~175,000 years ago, well before the split between the mexicana and parviglumis subspecies of teosinte and just before the split between Z. mays and Zea luxurians , using calculated nucleotide substitution rates for maize [21] and a calculated time since the split between mexicana and parviglumis of ~60,000 years and parviglumis and luxurians of ~140,000 years [22] . It will be interesting to test whether the Tcb1-male and Ga1-male genes diverged at a similar time, suggesting that the male–female genes were paired before divergence of Tcb1-s and Ga1-s . Tcb1-s and Ga1-s are mostly cross-incompatible with one another, suggesting the male genes are also divergent. However, Tcb1-s and Ga1-s are not fully cross-incompatible. In situations where pollen rejection is not absolute, Tcb1-s pollen has a competitive advantage over tcb1 pollen on Ga1-s or Ga2-s silks. This is true for all combinations of interactions between crossing barrier loci [7] , [12] and is consistent with them encoding related proteins. The confounding result that the behavior of pollen tubes during rejection by each system is slightly different may be explained by differences in amino acid sequence or differences in expression level or pattern between the haplotypes [4] . Tcb1-f/PME38 encodes a group 1 type of PME without an N-terminal pectin methylesterase inhibitor domain [23] , and contains a predicted signal peptide, so it has the potential to be secreted and interact directly with the pollen tube to remove methyl-esters from the pectin wall of the pollen tube. Esterified pectins are typically associated with the tip of the growing pollen tube, while de-esterified pectins are enriched distally, and there is a correlation between pectin de-esterification and increased cell wall stiffness [24] . Pollen cells finely tune the stiffness of the tip cell wall to sustain pollen tube elongation. Either under-supply or over-supply of PME activity can result in disturbed pollen tube growth and compromised male fertility [25] , [26] , [27] , [28] . The TCB1-F (and ZMPME3) protein falls into the Plant 1a clade of mature PME enzymes [29] (Supplementary Fig. 8 ). In summary, genetic and genomic data identify the Tcb1-female barrier gene as a PME38 homolog. Teosinte lines carrying Tcb1-f block maize pollen that lacks the male function provided by Tcb1-m . That the Tcb1-f gene encodes a cell wall modifying enzyme is consistent with the result that heterozygous Tcb1-s/tcb1 pollen is functional on Tcb1-s silks rather than active targeting of a pollen protein encoded by (a hypothetical maize allele of) the tcb1-m gene [11] . Surprisingly, it was shown that another PME family member is encoded by the Ga1-male gene [30] (in a very distinct clade, Plant X2, of PME enzymes (Supplementary Fig. 8 )), raising the possibility that the biochemical barrier to pollen and the ability of pollen to overcome that barrier are conferred by different classes of PME proteins. It will be interesting to test how universal this barrier mechanism is in sexual plant reproduction. The grasses also have an unusually high species diversity for a family with abiotic pollinators [31] . Identification of the Tcb1-female gene may facilitate research into the mechanisms of speciation in the grasses. Maize and teosinte lines and growth conditions All Tcb1-s lines used in this study have had the Tcb1-s haplotype introgressed from their maize or teosinte line of origin into standard maize lines W22 or B73 by backcrossing. The location of origin of these lines has been described elsewhere [4] , [7] , [8] , [10] . Plants were grown under summer field conditions at either Stanford, California or Madison, Wisconsin. Tcb1-s mapping As described before [7] , a Central Plateau teosinte collection 48703 [9] carrying the Tcb1-s barrier was backcrossed to the Mid-western US dent inbred W22 to incorporate the Tcb1-s locus into a maize background. This Tcb1-s strain was crossed to a chromosome 4 maize tester line virescent17 ( v17 ) brown midrib3 ( bm3 ) sugary1 ( su1 ), and the F1 was then backcrossed to the same tester line. Recombinants carrying crossovers between the four visual markers were tested for the Tcb1-s male and female functions in reciprocal crosses with Tcb1-s/su1 F1 plants. PCR mapping markers were developed to refine the location of crossovers in these recombinants. Tcb1-f knockout mutant screen To identify loss-of-function mutants of Tcb1-female , a Ga1-m Tcb1-s active Mutator strain was crossed to maize inbred A195 su1 ( tcb1 ), and then the progeny were grown as an open-pollinated block. Most of the progeny are expected to be heterozygous for Tcb1-s and su1 in repulsion with su1 ~6 cM away from the tcb1 locus [7] . Due to the rejection of the tcb1 pollen (which is predominantly su1 ), about 3% of the kernels in every ear with functional Tcb1-f are expected to be sugary in this open-pollinated population, while those without a crossing barrier were predicted to segregate su1 at 25%. Mixed pollination experiments For the mixed pollination testing of the two tcb1-f knockout mutants, two pollen donor lines and three pollen receiver lines were used. Pollen from a maize line ( tcb1 ) that does not have the Tcb1-s barrier genes but carries the endosperm color marker R1-self color ( R1-sc ) will produce purple kernels after fertilization of the lines used, while pollen from the knockout plants and the Tcb1-m plants carry r1-r and produce anthocyaninless kernels that are white or yellow. After being collected from the two donors and mixed, pollen was put on the three receiving ears: (1) a Tcb1-s tester ear was used to verify the presence of the Tcb1 male function from the tcb1-f::KO pollen; (2) the tcb1-f (KO) ear was used to test the presence/absence of the female barrier function in the knockout mutant; and (3) a maize ( tcb1 ) neutral ear was used to assay the percentage of viable pollen grains from the two donors in the mixture. Because any two tassels cannot be counted on to produce the same amounts of pollen, the ratio of the two pollen types in any mix cannot be assumed to be 1:1. Consequentially, it is essential to make a cross of each pollen mix onto a standard tcb1 maize ear (with a known pollen acceptance/function bias of 60% tcb1 : 40% Tcb1-s [10] ) to verify the ratio of functional pollen grains in the mix. The same protocol was used on the spontaneous Tcb1-m plant, except the Tcb1-m plant being tested was substituted for the KO plant. For mixed pollinations of the tcb1-f::silent lineage mop1 double-mutant plants, pollen from the same R1-sc tcb1 line and a r1-r Tcb1-s tester line was collected, mixed, and applied to the individual silent line ears and the neutral maize ears. Silk tissue collection, RNA isolation, and cDNA synthesis Plants for RNA isolation were grown in summer field conditions in Stanford, CA. Silk tissues were collected around 11 a.m., immediately put into liquid nitrogen in the field, and stored at −80 °C. Total RNA was isolated from silks with Trizol reagent (Invitrogen), DNase-treated, and either subjected to Illumina short read paired end RNA-seq, or used to synthesize the first strand cDNA with the Superscript IV RT kit (Invitrogen). Quantitative RT-PCR RT-PCR was performed on a Roche Lightcycler 480II (Roche Diagnostics). Each line/genotype had three biological replicates, and each in turn had three technical replicates. For cases where expression levels in individual plants is shown three technical replicates were used. Tubulin (Zm00001d033850) was used as a reference gene. In each line, relative expression levels were obtained by comparing Tcb1-f/PME38 to tubulin. 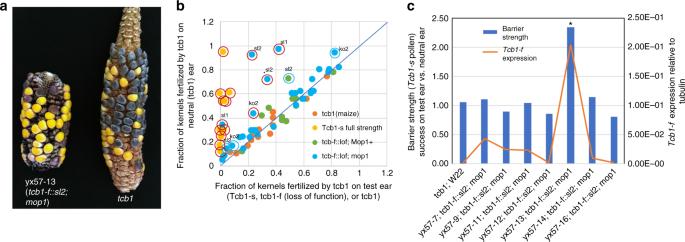Fig. 3 Reversion oftcb1-floss-of-function.aRevertant ear (marked by asterisk inbandc) pollinated by a mix oftcb1; R1-scandTcb1-m;r1pollen showing higher frequency of yellow kernels on the test ear than thetcb1control ear.bResults of mixed pollination tests on four genotypes:tcb1,Tcb1-s,tcb1-f(loss-of-function(lof))alleles, andtcb1-f(lof) mop1double mutants. The percentage of kernels fromtcb1pollen on the test ear are plotted on thex-axis and the percentage of kernels fromtcb1pollen on the controltcb1ear on they-axis. Equal percentages in the two ears indicates no barrier (line with slope = 1). Red circles indicate ears with significantly fewertcb1kernels in the test ear vs. the control ear atp< 0.0001 and blue circles at 0.0001 <p< 0.01 (two-tailed Fisher exact test). The loss-of-function line is indicated for each revertant.cTcb1-f/PME38gene expression level and barrier strength. Barrier strength is expressed as the ratio of kernels fromTcb1-svs.tcb1pollen on the test ear vs. the controltcb1ear (columns), with a fraction of 1.0 indicating no barrier and significantly higher values a functional barrier.Tcb1-f/PME38RNA levels are expressed as relative to thetubulincontrol gene (orange line). Error bars incequal the standard error of the mean. Individual pedigree numbers are given for loss-of-function plants tested for reversion inaandc. Source data for panelsbandcis provided in a Source Data file 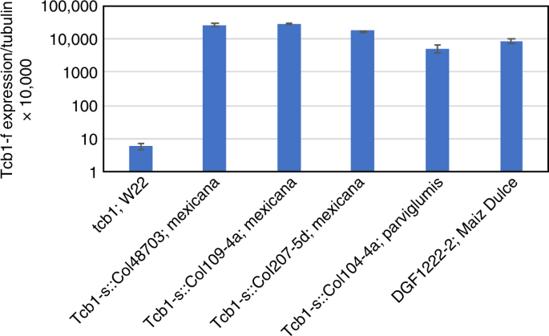Fig. 4 Mean expression ofTcb1-f/PME38in lines with differentTcb1-shaplotypes. W22 is a standard maizetcb1line,Tcb1-s::Col48703,Tcb1-s::Col109-4a, andTcb1-s::Col207-5dare three independent collections ofZea maysssp.mexicanatesointe lines;Tcb1-s::Col104-4a, aZea maysssp.parviglumisline; and DGF1222-2 derived from Maiz Dulce, an ancient Mexican maize sweet corn variety8. Error bars equal the standard error of the mean. Source data for RT-PCR are provided as a Source Data file Primers are listed in Supplementary Table 3 . Sequencing, assembly, and analysis All the RNA and DNA sequencing works were done with Illumina Paired-end sequencing by Novogene (CA, USA). RNA-seq reads from all samples were combined and de novo assembled with Trinity v2.4.0 [32] . The gene in contig DN33598_c7_g3_i1 was identified as the Tcb1-f candidate gene due to its extremely high expression in the functional Tcb1-s line and the near lack of expression in the KO mutants and a standard W22 maize line. PCR primers were designed based on the DN33598_c7_g3_i1 sequence, and one BAC clone was isolated from a library made from a maize line into which the Tcb1-s::Col48703 haplotype had been introgressed. The BAC sequencing reads were assembled with SPAdes v3.11.1 [33] . NODE_62, a contig that is 13,656 bp with coverage of 4029, was identified as having the Tcb1-f candidate gene. Whole genome sequencing reads from the two KO mutants were individually assembled with SPAdes v3.11.1 and BLASTed against NODE_62. Also, the mutant sequencing reads were mapped against NODE_62 using GSNAP [34] . Combining both approaches identified the hopscotch retrotransposon insertion in the tcb1-f(KO1)- mutant allele. For phylogenetic analyses, alignments were made using the ClustalW algorithm in MegAlign (DNASTAR). The predicted mature PME enzymes and the Arabidopsis PME family members were taken from Markovic and Janecek, as were the subfamily designations [29] . Phylogenies were produced from these alignments using MrBayes v3.2.0 using default settings for amino acid analysis [35] . The MrBayes analysis was performed for 4,100,000 generations at which point the standard deviation of the split frequencies was below 0.004. Reporting summary Further information on research design is available in the Nature Research Reporting Summary linked to this article.